Accelerated discovery of cathode materials with prolonged cycle life for lithium-ion battery Large-scale battery systems are essential for efficiently utilizing renewable energy power sources from solar and wind, which can generate electricity only intermittently. The use of lithium-ion batteries to store the generated energy is one solution. A long cycle life is critical for lithium-ion battery when used in these applications; this is different from portable devices which require 1,000 cycles at most. Here we demonstrate a novel co-substituted lithium iron phosphate cathode with estimated 70%-capacity retention of 25,000 cycles. This is found by exploring a wide chemical compositional space using density functional theory calculations. Relative volume change of a compound between fully lithiated and delithiated conditions is used as the descriptor for the cycle life. On the basis of the results of the screening, synthesis of selected materials is targeted. Single-phase samples with the required chemical composition are successfully made by an epoxide-mediated sol–gel method. The optimized materials show excellent cycle-life performance as lithium-ion battery cathodes. Among the range of lithium-ion battery (LIB) cathode materials, LiFePO 4 (LFP) has advantages in cost, safety and cycle life as compared with others [1] , [2] . When renewable energy-storage applications are considered, however, the cycle life of LFP needs to be further improved. Cycle life is typically defined as the number of complete charge/discharge cycles before its capacity falls down to a certain level, say 70%, of its initial value. Our target of the long-life battery is more than 70% capacity retention after 10,000 cycles. If this target is met then LIB can meet the lifetime cost requirement for their use over 30 years with a daily charge/discharge cycle. The present study aims to develop LFP materials that exhibit prolonged cycle lives by substituting a range of solute elements on the different cation sites of the LFP material. The selection of suitable solute elements is labour-intensive for two reasons. First, the exploration space is huge when multiple solute elements and a variety of chemical compositions are considered. Second, many different metastable phases often appear depending upon the synthesis and processing conditions, such as synthesis temperature, synthesis routes and so on, even when the chemical composition is fixed. A clear idea of which phase to be targeted is essential before starting the actual synthesis experiments. Discovery of and optimization of materials for a particular application has often been achieved by chance after lengthy trial-and-error iterations, neither by rational exploration of the whole chemical compositional space, nor on the basis of clear design principles. Recently, challenges for accelerated discovery of materials with the aid of information technology have been demonstrated [3] . One of the approaches uses high-throughput screening of material database that is generated by first principles density functional theory (DFT) calculations [4] , [5] , [6] . Thanks to the recent progress of computational power and techniques, a large number of DFT calculations can be performed with the accuracy comparable to experiments. This can be used for high-efficiency material exploration. Another approach is based upon state-of-the-art machine-learning algorithms to search the optimum in the chemical compositional space [7] . A combined approach of both techniques has also been used [8] , [9] . The cycle life of LIB cathodes is not a quantity that can be derived by a simple physical model. It is determined by the degradation rate during repeated charge/discharge cycles that is influenced by many different factors. The charge and discharge processes for LFP proceeds via a two-phase reaction, and which inevitably produces interphase boundaries with different lattice parameters [10] . The volume change of crystalline lattice between LFP and fully delithiated FP is 6.5% [1] . Microcracks are often formed because of the stress inside the LFP cathodes during the repeated charge/discharge cycle, which is widely accepted as the major degradation mechanism of the LFP cathode [11] . The degradation could therefore be retarded by reducing the volume change of the crystalline lattice during the charge/discharge cycle. Here we assume that the relative volume change (RVC) of a compound between fully lithiated and delithiated conditions can be used as the descriptor for the cycle life. We then explore a wide chemical compositional space in order to optimize solute atoms in LFP cathode materials for prolonged LIB cycle life by systematic DFT calculations. On the basis of the results of the screening, synthesis of selected materials can be targeted. After synthesis of single-phase samples with the required chemical composition, excellent cycle-life performance as LIB cathode is confirmed. Systematic DFT calculations In the present study, a large set of DFT calculations is systematically made for many different kinds of solute elements that are substituted on three possible cation sites of LFP. Many experimental and theoretical studies on solute atoms in LFP have been reported since the early work of the aliovalent doping in LFP [12] . There has been controversy on the capability of the aliovalent doping. History of the debate on the doping can be found in reference [13] . It should be emphasized that they discussed the solubility of single aliovalent dopants and related defect/carrier formation in LFP. The situation is very different from the present study where we treat only co-substitution of elements to maintain the charge neutrality within the compound. Generally speaking, single aliovalent elements and co-substitution of elements behave differently in wide-gap materials. In the present study, the charge neutrality is maintained by assuming that the formal ionic charges are unchanged. For example, when Zr 4+ and Si 4+ are incorporated and are located, respectively, at Fe 2+ and P 5+ sites, two Si atoms and one Zr atom are put into the supercell of the DFT calculation. The situation can be expressed as (Zr Fe +2 Si P ). The chemical compositional space investigated in the present study is shown as 630 cubes in Fig. 1a . DFT calculations are thoroughly made for all possible solute arrangements within the unit cell composed of four formula units of LFP (that is, 28 atoms). The lowest energy structure among them is adopted as the one representing the given chemical composition. An example of the dependence of the energy on the solute arrangement is shown in Fig. 1b . A section of the results obtained from the calculations for the relative volume change between lithiated and fully delithiated materials is shown in Fig. 1a . RVC is defined by 100·( V L – V D )/ V L (%), where V L and V D denote lattice volumes of lithiated and delithiated material LFP, respectively. 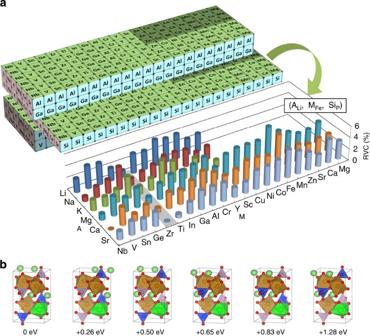Figure 1: Theoretical results of co-substituted LFP. (a) Variety of the chemical compositional space investigated in the present study. The shaded area corresponds to chemical compositions that are excluded from the present study, since the charge compensation is not possible within the given supercell. Calculated RVC between lithiated and fully delithiated materials on a (ALi, MFe, SiP) section is shown together. (b) An example of the dependence of the energy on the solute arrangements for (LiLi, ZrFe, SiP), that is, Z2S material. The energy is per four formula units of LFP, and relative to the lowest energy arrangement. Orange and green octahedrons, respectively, denote FeO6and ZrO6. Violet and blue tetrahedrons denote PO4and SiO4, respectively. Green and red balls, respectively, show Li and O. Figure 1: Theoretical results of co-substituted LFP. ( a ) Variety of the chemical compositional space investigated in the present study. The shaded area corresponds to chemical compositions that are excluded from the present study, since the charge compensation is not possible within the given supercell. Calculated RVC between lithiated and fully delithiated materials on a (A Li , M Fe , Si P ) section is shown together. ( b ) An example of the dependence of the energy on the solute arrangements for (Li Li , Zr Fe , Si P ), that is, Z2S material. The energy is per four formula units of LFP, and relative to the lowest energy arrangement. Orange and green octahedrons, respectively, denote FeO 6 and ZrO 6 . Violet and blue tetrahedrons denote PO 4 and SiO 4 , respectively. Green and red balls, respectively, show Li and O. Full size image According to the series of calculations performed, the effective ways of reducing the RVC are found by double substitutions of LFP with either Si 4+ or Al 3+ at the P site and trivalent or tetravalent cations at the Fe site. Among them, some sets of substitutions show RVC of smaller than 3%: for example, (Y Fe +Si P ), (Zr Fe +2 Si P ) and (Zr Fe +Al P ). We will focus on the (Zr Fe +2 Si P ) system, which will be hereafter called Z2S. Its chemical formula is Li(Fe 1− x Zr x )(P 1−2 x Si 2 x )O 4 . DFT calculations for Z2S with supercells composed of 8 and 16 formula units are additionally made, which corresponds to x =0.125 and 0.0625, respectively. Results of the RVC are shown in Fig. 2(a) together with the trends observed in the mismatch of the (100) planes (bc planes) between lithiated and delithiated materials ( Fig. 2b) . The planar mismatch is defined by 100·( A L – A D )/ A L (%), where A L and A D denote areas of bc planes in lithiated and delithiated materials, respectively. According to the domino-cascade model by Delmas et al. [10] for the delithiation mechanism of LFP, the interphase boundaries between LFP and FP prefer (100) planes. A smaller planar mismatch between the planes is therefore expected to be beneficial for retarding the degradation during repeated charge/discharge cycles. 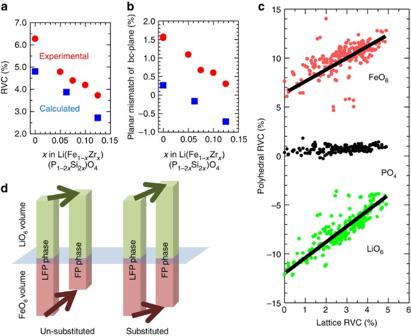Figure 2: Effects of solutes on RVC. (a) RVC between lithiated (δ=0) and delithiated (δ=1−x) materials for Li1−δ(Fe1−xZrx)(P1−2xSi2x)O4. Blue square and red circle denote DFT results and experimental results, respectively. (b) Planar mismatch of (100) planes (bc planes) between lithiated and fully delithiated materials for Li1−δ(Fe1−xZrx)(P1−2xSi2x)O4. (c) Correlations between the RVC of FeO6, LiO6and PO4polyhedra with the lattice RVC for many different substituted materials. (d) Explanation of the solute effects on the lattice RVC. Figure 2: Effects of solutes on RVC. ( a ) RVC between lithiated ( δ =0) and delithiated ( δ =1− x ) materials for Li 1−δ (Fe 1− x Zr x )(P 1−2 x Si 2 x )O 4 . Blue square and red circle denote DFT results and experimental results, respectively. ( b ) Planar mismatch of (100) planes (bc planes) between lithiated and fully delithiated materials for Li 1−δ (Fe 1− x Zr x )(P 1−2 x Si 2 x )O 4 . ( c ) Correlations between the RVC of FeO 6 , LiO 6 and PO 4 polyhedra with the lattice RVC for many different substituted materials. ( d ) Explanation of the solute effects on the lattice RVC. Full size image Both the volume and the planar mismatch decrease linearly with the solute concentration. A possible mechanism for the decrease in the RVC following the substitutions is briefly discussed here. Figure 2c shows correlations between the RVC of FeO 6 , LiO 6 and PO 4 polyhedra with the lattice RVC for many different substituted materials that have been calculated in the present study. A clear trend can be seen between the lattice RVC and the polyhedral RVC for FeO 6 and LiO 6 . On the other hand, the polyhedral RVC for PO 4 is almost unaffected by the lattice RVC. The magnitude of the reduction of the polyhedral RVC is larger in LiO 6 than in FeO 6 , which explains the observed effect with the substituted LFP. As drawn in Fig. 2d , the polyhedral RVC became smaller in FeO 6 and larger in LiO 6 in the substituted LFP, thereby making the lattice RVC smaller. Synthesis and characterization of targeted materials On the basis of the results of the computational screening of the substituted LFP, synthesis experiments were performed for Li(Fe 1− x Zr x )(P 1−2 x Si 2 x )O 4 materials with varying x . Initially, the conventional solid-state reaction method was used. Many different procedures, starting materials, synthesis temperatures, atmospheres and durations were tried; however, the production of a single-phase solid-solution material was unsuccessful. We have chosen to use an epoxide-mediated sol–gel method to obtain more intimate mixing of the starting materials. By optimizing the processing parameters, single-phase solid-solution samples were successfully synthesized. Pictures of the sol–gel products and the final powder sample are shown in Fig. 3a,b . Particle diameters using scanning electron microscopy were ~0.1 μm in both pristine and co-substituted samples. 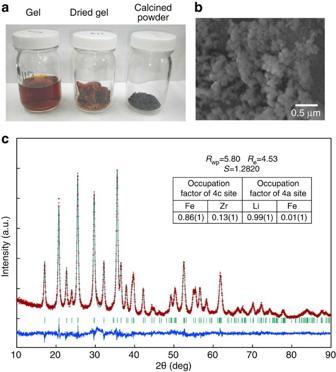Figure 3: Synthesis of Z2S co-substituted LFP. (a) Pictures of the gel, dried gel and the final calcined powder for the Li(Fe1−xZrx)(P1−2xSi2x)O4sample withx=0.125. (b) Scanning electron microscopy image of the calcined powder withx=0.125. (c) XRD (Cu-Kα) profile and the result of the Rietveld refinement for the Li(Fe1−xZrx)(P1−2xSi2x)O4sample withx=0.125. Figure 3: Synthesis of Z2S co-substituted LFP. ( a ) Pictures of the gel, dried gel and the final calcined powder for the Li(Fe 1− x Zr x )(P 1−2 x Si 2 x )O 4 sample with x =0.125. ( b ) Scanning electron microscopy image of the calcined powder with x =0.125. ( c ) XRD (Cu-Kα) profile and the result of the Rietveld refinement for the Li(Fe 1− x Zr x )(P 1−2 x Si 2 x )O 4 sample with x =0.125. Full size image Structural analysis by the powder X-ray diffraction (XRD) shows that the samples of Li(Fe 1− x Zr x )(P 1−2 x Si 2 x )O 4 are single-phase up to the value of x =0.125. XRD patterns are shown in Supplementary Fig. 1 . Figure 3c shows the result of the Rietveld refinement [14] of the XRD profile for the x =0.125 sample. Only 1% of the Li site is found to be occupied by Fe and the Zr content at the Fe site is 13%, which satisfactorily agrees to the intended ratio of cations and the mixed quantities. We can therefore conclude that single-phase solid-solution samples of Z2S are successfully synthesized up to x =0.125. More details of the XRD analyses were described in Supplementary Note 1 . Electrochemical experiments We first made experiments using a beaker-type cell with a lithium metal anode. Charge and discharge curves with the Z2S ( x =0.125) cathode and the rate of 170 mAg −1 (corresponding to 1C for the pristine cathode) are shown in Fig. 4a . First discharge capacity was 128 mAhg −1 , which corresponds to 88% of theoretical capacity (145 mAhg −1 for Z2S ( x =0.125) cathode). The cells with the pristine and the Z2S ( x =0.125) cathodes are compared in Supplementary Fig. 2 of Supplementary Note 2 . Both of them exhibit a plateau at the same potential value, 3.4 V, implying that the co-substitution does not affect the redox reaction of Fe ions significantly. Their rate capabilities are found to be almost the same. 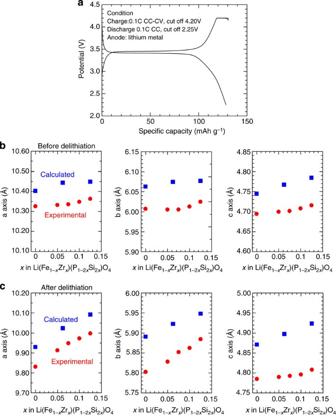Figure 4: Charge/discharge experiments with Z2S cathodes. (a) Charge and discharge curves for a beaker-type cell with Li(Fe1−xZrx)(P1−2xSi2x)O4cathode ofx=0.125. (b) Experimental and calculated lattice parameters of Z2S samples as a function of the solute concentration before delithiation and (c) after delithiation. Red circles and blue squares correspond to experimental and calculated results, respectively. Figure 4: Charge/discharge experiments with Z2S cathodes. ( a ) Charge and discharge curves for a beaker-type cell with Li(Fe 1− x Zr x )(P 1−2 x Si 2 x )O 4 cathode of x =0.125. ( b ) Experimental and calculated lattice parameters of Z2S samples as a function of the solute concentration before delithiation and ( c ) after delithiation. Red circles and blue squares correspond to experimental and calculated results, respectively. Full size image The experimental and calculated lattice parameters of compounds before and after the delithiation are shown in Fig. 4b,c as a function of solute concentration, x . The lattice parameters for all three axes show small dependence on x before the delithiation. The dependence is much larger in the delithiated compounds especially for a and b axes. In other words, the presence of the solute elements has a much larger impact on the structure of delithiated compounds. The experimental lattice RVC and the planar mismatch of bc plane are shown in Fig. 2a,b to compare with the computed values. Satisfactory agreements between experiments and computed results can be seen. The experimental lattice RVC decreases linearly with x from 6.3% ( x =0) to 3.7% ( x =0.125). A similar trend can be observed for the planar mismatch of bc planes. It decreases linearly with x from 1.5% ( x =0) to 0.3% ( x =0.125) by experiments. We can therefore expect that the strain energy at the interphase boundary of LFP/FP can be significantly decreased by the co-substitution of LFP. The cycle life performance was examined for the Z2S cathode in an aluminium-laminated pouch cell using a natural graphite anode. A cell with a pristine LFP cathode was prepared for comparison. Charge/discharge cycles of the cells were made between 2.00 and 3.80 V using a 1 C current rate. The specific capacity of two cells with Z2S ( x =0.050) cathode (Cell-A) and pristine cathode (Cell-B) are compared in Fig. 5a . Although the initial capacity of Cell-B with pristine LFP cathode (144 mAh g −1 ) was higher than that of Cell-A (125 mAh g −1 ), the capacity fades much faster in Cell-B. As a result, the capacity became larger in Cell-A after 2,100 cycles. The cycle life with 80% capacity retention was 10,000 cycles for Cell-A, whereas it was 1,800 cycles for Cell-B. This significant increase in cycle life of Cell-A compared with Cell-B can be ascribed to the difference in the cathodes, since all other components of the cell and cell testing are the same. The capacity retention often shows linear decrease with the square root of the number of cycles. Using this empirical relationship, the cycle life observed for 70% capacity retention can be estimated as 25,000 cycles for Cell-A. This is significantly greater than our target cycle life of 70% capacity retention of 10,000 cycles. It should be noted that the substitution of Fe by Zr inevitably decreases the theoretical capacity because Zr cannot contribute to the redox reaction under the present condition. However, initial capacity of cathode is not the critical parameter for the large-scale battery systems, contrary to the application to portable devices. The capacity after many cycles, as the result of large initial capacity and slow capacity fading, is crucial. 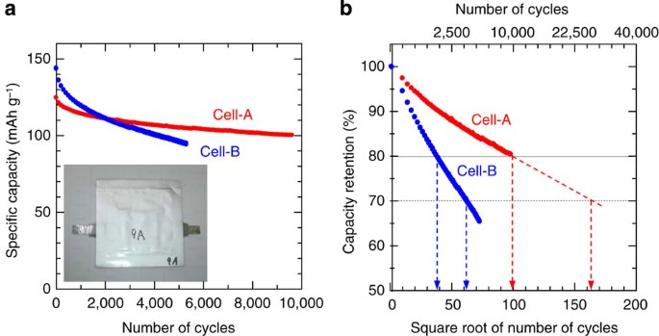Figure 5: Cycle life experiments with Z2S cathode. (a) The specific capacity of two pouch cells with pristine and Z2S (x=0.050) cathodes as a function of number of charge/discharge cycles. An inset photo shows an aluminum-laminate pouch cell used for the cycle-life performance tests. (b) The capacity retention plotted against the square root of the number of cycles. Red and blue circles correspond to Cell-A and -B, respectively. Figure 5: Cycle life experiments with Z2S cathode. ( a ) The specific capacity of two pouch cells with pristine and Z2S ( x =0.050) cathodes as a function of number of charge/discharge cycles. An inset photo shows an aluminum-laminate pouch cell used for the cycle-life performance tests. ( b ) The capacity retention plotted against the square root of the number of cycles. Red and blue circles correspond to Cell-A and -B, respectively. Full size image We have rationally explored a wide chemical compositional space for co-substituted LFP in order to optimize LFP cathode materials for prolonged LIB cycle life. Systematic DFT calculations were performed for a wide range of substituted LFP and FP materials. It was predicted that concurrently substituting LFP on the Fe and P sites with Zr and Si, respectively, by x =0.125 reduced the lattice RVC by 40%; this was verified experimentally. The observed planar mismatch of bc planes of the substituted samples was as low as 0.3%, which was significantly smaller than that of the pristine sample, 1.5%. Electrochemical tests found that the rate capability of the cell with the co-substituted LFP was almost the same as that with the pristine LFP. The cycle life tests performed in a full cell configuration with a graphite anode showed that the cycle life of the cell containing the optimized Z2S ( x =0.050) cathode outperforms the cell containing the standard pristine cathode by a factor of 5, and the estimated cycle life for 70% capacity retention was 25,000 cycles. This approach of screening materials using a large set of DFT is useful for the exploration of a large chemical compositional space. Accelerated discovery of suitable materials can therefore be performed and specific compositions can be targeted to confirm the results experimentally. First-principles calculations Calculations were made for all possible solute arrangements within the unit cell composed of four formula units (28 atoms for LFP). As for the substituted LFP, one of the four Li atoms in the unit cell was substituted by cations of six elements (Li + , Na + , K + , Mg 2+ , Ca 2+ , Sr 2+ ). One of the four Fe atoms was substituted by cations of 21 elements (Mg 2+ , Ca 2+ , Sr 2+ , Mn 2+ , Fe 2+ , Co 2+ , Ni 2+ , Cu 2+ , Zn 2+ , Sc 3+ , Y 3+ , Cr 3+ , Al 3+ , Ga 3+ , In 3+ , Ti 4+ , Zr 4+ , Ge 4+ , Sn 4+ , V 5+ , Nb 5+ ). P was substituted by cations of five elements (Al 3+ , Ga 3+ , Si 4+ , P 5+ , V 5+ ). The number of the substituted atoms was determined so that the formal charge of Fe is +2. The delithiated states were constructed by removing Li atoms. The maximum number of removed Li atoms was determined so that the formal charge of Fe was at most +3 and those of the other elements were unchanged. All possible arrangements of the solute atoms were examined within the unit cell, and the most stable arrangement was selected to estimate the lattice constants for each set of the solute elements. The total number of DFT calculations was ~2,000. First-principles DFT calculations were performed using the plane-wave basis projector-augmented wave method implemented in VASP code [15] . The plane-wave basis set was determined with a cutoff energy of 400 eV for initial screening ( Fig. 1 ). Additional calculations shown in Figs 2 and 4 were made with the cutoff energy of 500 eV. Integral in the reciprocal space was evaluated by the Gaussian smearing technique with a smearing parameter of 0.1 eV and a 2 × 3 × 3 mesh. Spin polarization was considered assuming collinear and parallel magnetic structures. The exchange-correlation interaction was treated by the generalized gradient approximation [16] with the Hubbard model correction (GGA+ U ) [17] . We used U -parameters of 2, 2, 3, 4, 4, 4 and 5 eV for Ti, V, Cr, Mn, Fe, Co and Ni, respectively. The U -parameters were not used for the rest of the elements. Atomic positions and lattice constants were optimized until the residual forces and stresses, respectively, became smaller than 0.02 eV/Å and 2 GPa for the initial screening ( Fig. 1 ), and 0.02 eV/Å and 0.2 GPa for the additional calculations ( Figs 2 and 4 ). Sol–gel synthesis Samples were prepared by using the sol–gel possessing mediated by epoxides [18] , [19] . A conclusive advantage of the epoxide-mediated technique is that it allows the use of common metal salts as the sol–gel precursors, eliminating the need for highly reactive metal alkoxides. This technique has also proven to be useful in designing the precursor gels of highly homogensous complex oxides [20] , [21] , [22] , [23] . In this study, lithium acetate (CH 3 COOLi), iron nitrate nonahydrate (Fe(NO 3 ) 3 ˙9 H 2 O), zirconium chloride (ZrCl 4 ), tetraethyl orthosilicate (Si(OC 2 H 5 ) 4 ) and phosphoric acid (H 3 PO 4 ) were used as the sources of inorganic components, and ethanol was used as the solvent. Propylene oxide (PO) was added as a proton scavenger to promote gelation. All the reactants and solvents were reagent grade and were used as received. The typical molar ratio in the starting composition was CH 3 COOLi: Fe(NO 3 ) 3 ·9 H 2 O: ZrCl 4 : Si(OC 2 H 5 ) 4 : H 3 PO 4 : ethanol: PO=1: 1− x : x : 2 x : 1−2 x : 26.7: 27 so as to fabricate samples with the composition of Li(Fe 1− x Zr x )(P 1−2 x Si 2 x )O 4 upon calcination. The samples were prepared as follows. First, the cation sources were dissolved into ethanol under ambient atmosphere to give a homogeneous solution. Then, PO was added dropwise to the transparent solution under stirring. After that, the resultant solution was allowed to gel in a closed container at 40 ° C for 24 h, and the wet gel was dried at 40 ° C. The dried gel was ground in a mortar and calcined at 550 ° C for 12 h under nitrogen atmosphere. Scanning electron microscopy observation of the final products found that the particle diameters were ~0.1 μm for all samples. XRD refinements Rietveld refinements [14] were made for Z2S samples with a constriction that Si substitutes only P because Si is most likely to take only fourfold coordination. The occupation factors of 4a (Li site) and 4c (Fe site) were then determined. Since the occupation factor for Li at 4a was close to unity, factors for Fe and Zr at 4a were indistinguishable. The occupation factor for Li at 4c was not able to be resolved, either. Electrochemical tests A beaker-type three-electrode cell was used for the delithiation. The working electrode was fabricated by mixing of the cathode powder, electronic conductor and binder at a ratio of 100:10:10 by weight. Acetylene black (Denkikagaku Kogyo) was used for the electronic conductor, and polyvinylidene difluoride (PVdF, Kureha) was used for the binder. In order to make the electrode, the mixture was dissolved in N -methyl pyrrolidone, and then cast on aluminium foil of 20 μm thick. The electrode was dried at 80 ° C in air and pressed to increase the electrode density. Lithium metal foil was used for the counter and reference electrodes. The electrolyte was a 1 M solution of LiPF 6 in mixture of ethylene carbonate (EC) and dimethyl carbonate (DMC) with a 2:1 volume ratio (LBG-00938 LiPF 6 , EC/DMC, Kishida Chemical Corp., Ltd.). Charge and discharge were carried out at 0.1C rate between 2.25 V as the lower limit and 4.20 V as the upper limit at the constant temperature of 25 ° C. 1C is defined as 170 mA g −1 for all samples for simplicity. An aluminium-laminate pouch cell was used for cycle-life performance tests. The cathode was fabricated by the same procedures as mentioned above. The electrode was cut into 20 mm × 20 mm square sheet and aluminium leads (50 mm × 5 mm × 0.1 mm) were welded as cathode leads. The mixture of a natural graphite (Hitachi Chemical) and binder (PVdF, Kureha) was dissolved in N -methyl pyrrolidone at the ratio of 100:10, and then cast on 12 μm of copper foil. The electrode was dried at 80 ° C in air and pressed to increase the electrode density. This anode electrode was cut into 22 mm × 22 mm square sheet and nickel leads (50 mm × 5 mm × 0.1 mm) were welded as anode leads. The cathode electrode, a polypropylene separator (Celgard, Polypore) and anode electrode were stacked and then put into an aluminium-laminate pouch. The electrolyte as mentioned above was poured into the aluminium-laminate pouch. This pouch was sealed using vacuum sealer to avoid permeation of moisture. Charge and discharge were carried out at 1C rate between 2.00 V as the lower limit and 3.80 V as the upper limit at the constant temperature of 25 ° C. 0.1 C charge and discharge were also carried out every 100 cycles to measure the capacity retention. How to cite this article : Nishijima, M. et al. Accelerated discovery of cathode materials with prolonged cycle life for lithium-ion battery. Nat. Commun. 5:4553 doi: 10.1038/ncomms5553 (2014).